Molecular decoding using luminescence from an entangled porous framework Chemosensors detect a single target molecule from among several molecules, but cannot differentiate targets from one another. In this study, we report a molecular decoding strategy in which a single host domain accommodates a class of molecules and distinguishes between them with a corresponding readout. We synthesized the decoding host by embedding naphthalenediimide into the scaffold of an entangled porous framework that exhibited structural dynamics due to the dislocation of two chemically non-interconnected frameworks. An intense turn-on emission was observed on incorporation of a class of aromatic compounds, and the resulting luminescent colour was dependent on the chemical substituent of the aromatic guest. This unprecedented chemoresponsive, multicolour luminescence originates from an enhanced naphthalenediimide–aromatic guest interaction because of the induced-fit structural transformation of the entangled framework. We demonstrate that the cooperative structural transition in mesoscopic crystal domains results in a nonlinear sensor response to the guest concentration. Distinguishing small structural differences in molecules is a critical and challenging task for applications in biotechnology, environmental monitoring, gas separation and molecular sensor design. In particular, a key principle for the fabrication of chemosensors is that they must be able to detect differences in explosive, harmful or polluting small molecules, and sequentially implement a recognition–transduction protocol ( Fig. 1a ) [1] , [2] , [3] , [4] . This recognition should selectively trap specific molecules, and the transduction should convert the recognition event into a detectable signal. A general strategy for increasing selectivity includes enhancing the level of sophistication in the recognition unit for a target molecule by optimizing the host–guest interaction, or simply stated, by arraying various hosts to produce a composite response that is unique to each analyte, known as 'an electronic nose' [5] . However, these systems require a number of host matrices for the selective sensing of a specific molecule. In this study, we propose a molecular decoding methodology to provide a single host domain that accommodates several chemically diverse analytes that can also differentiate between them by transducing a particular host–guest interaction into a corresponding readout ( Fig. 1b ). The key to success in this process involved the use of an innovative transduction mechanism that directly visualizes the host–guest interaction itself, which corresponds to the intrinsic nature of the guest analyte. 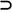Table 1 Properties of1VOCs. No description available Figure 1: Conventional molecular sensing and molecular decoding protocols. ( a ) The conventional molecular sensing protocol is demonstrated by molecules or organic polymers that possess the following two distinct chemical units: a recognition part and a transduction part. An improvement in the recognition selectivity leads to a high sensing capability. ( b ) Molecular decoding materials can not only accommodate chemically diverse analytes but also differentiate between them by displaying a signal that corresponds to each analyte. The direct transduction of the host–guest interaction into a corresponding signal is key to the implementation of successful molecular decoding. Full size image Porous coordination polymers (PCPs) [6] , [7] , [8] , [9] , [10] , [11] , [12] , [13] , [14] , [15] , [16] , [17] with three-dimensional molecular skeletons that are assembled by organic linkers and inorganic joints can provide host matrices for molecular decoders. This arises from the inherent confinement effect within their nanopores, which enhances the host framework–guest interaction [18] , [19] , and the pore surface designability that enables the incorporation of an appropriate decoding unit into a scaffold through the use of strategic organic chemistry [20] , [21] . We designed an entangled framework, one of the most characteristic structural features of PCPs, from the elongation of organic linkers that lead to the intergrowth of one framework into the other, resulting in the catenation of the frameworks [22] , [23] . The entanglement of two chemically non-interconnected frameworks provides the dynamics from the dislocation of their mutual positions [24] . This entanglement dynamics of PCPs contribute to a decoding system as a result of the implementation of two processes. The first includes an induced-fit-type structural transformation that enables the entrapment of a variety of guest molecules by changing the pore size and shape to maximize the host–guest interaction ( Fig. 2a ). The second consists of a cooperative accommodation process due to the ordered structure of the mesoscopic crystal domains, which allows guest molecules simultaneous access to the decoding units and results in a nonlinear sensor response ( Fig. 2b ). 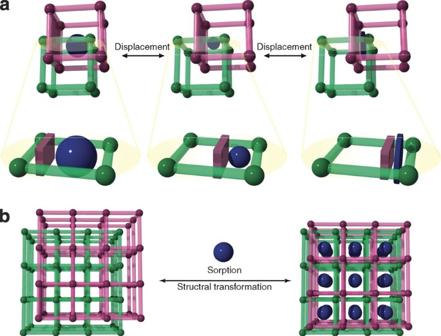Figure 2: Advantages of entangled PCPs for molecular decoding. (a) The framework entanglements provide flexibility through spaces when the pore size and shape are altered in response to the structure of a target guest molecule without changing the total void space. Chemically non-interconnected frameworks show dynamic movement by the dislocation of their mutual positions to effectively trap molecules while maximizing their host–guest interaction. (b) The crystallinity of an entangled framework ordered on the mesoscopic scale demonstrates a cooperative structural transition in response to guest accommodation in its crystal domain. This leads to simultaneous access to the decoding unit. Figure 2: Advantages of entangled PCPs for molecular decoding. ( a ) The framework entanglements provide flexibility through spaces when the pore size and shape are altered in response to the structure of a target guest molecule without changing the total void space. Chemically non-interconnected frameworks show dynamic movement by the dislocation of their mutual positions to effectively trap molecules while maximizing their host–guest interaction. ( b ) The crystallinity of an entangled framework ordered on the mesoscopic scale demonstrates a cooperative structural transition in response to guest accommodation in its crystal domain. This leads to simultaneous access to the decoding unit. Full size image Among several transduction techniques based on host–guest chemistry, such as optical, electrical, quartz crystal microbalance and surface acoustic wave techniques, luminescence is a highly sensitive and simple optical transduction method. This method does not require extensive hardware; the intensity of the luminescence is strong enough to be detected by the naked eye. In particular, luminescence, with a turn-on switching property that is triggered by a guest molecule, is intrinsically more sensitive than the more common luminescence-quenching method because detection occurs relative to a dark background. Although there have been a number of reports on luminescent PCPs [25] , and a few on guest-dependent luminescence [26] , [27] , [28] , [29] , none of the approaches thus far have demonstrated a plain distinguishable emission for each guest molecule, turn-on switching properties or a sensing capability for vapourized analytes. In this paper, we report on a 1,4,5,8-naphthalenediimide (NDI)-based entangled PCP that undergoes a dynamic structural transformation to confine a class of aromatic volatile organic compounds (VOCs), or tropospheric air pollutants [30] , [31] , and decodes the chemical substitution information of the aromatic species into recognizable photoluminescence in the visible light region. The aromatic species benzene, toluene, xylene, anisole and iodobenzene were indicated as blue, cyan, green, yellow and red, respectively. We show that this unusually wide range of emission arises directly from the enhanced NDI–VOC interaction that generates either exciplex fluorescence with charge transfer (CT) characteristics or phosphorescence stabilized by the heavy atom effect. These emission wavelengths are not only reasonably separated from each other but their intensity is also sufficiently amplified to be detected by the naked eye, whereas the framework without VOCs is not emissive. On the basis of this turn-on switching property, these sensors show a nonlinear luminescence response to VOC vapour concentration, with a higher sensitivity in the VOC lower-vapour-pressure region. Structural dynamics in response to guest accommodation The design principle used for the decoding unit involved incorporating a photoactive organic module, NDI [32] , [33] , into the porous framework as a scaffold because of its desirable characteristic photophysical properties. Despite its very low fluorescent quantum yield ( Φ f ∼ 0.003), NDI interacts with aromatic VOCs and generates an exciplex emission with CT characteristics, resulting in the production of a new weak fluorescence band ( Φ f <0.02) (ref. 34 ). We selected an entangled framework with a twofold interpenetration, [M 2 (dicarboxylate) 2 (amine)] n (refs 35 , 36 , 37 , 38 , 39 , 40 ), in which the dimetal joint is connected by four layers of dicarboxylate units and two pillar amine linkers. These connections form a three-dimensional framework with a primitive cubic topology, followed by catenation of the two frameworks ( Fig. 3 ). The decoding unit can be embedded into the framework scaffold as the pillar linker by simply incorporating the dipyridyl derivative of NDI. Structural determination is essential in elucidating the interaction between NDI and a guest molecule. We used single-crystal X-ray crystallography to reveal the manner in which the structural dynamics contribute to the efficient accommodation of guest molecules and to the optimization of host–guest interaction. 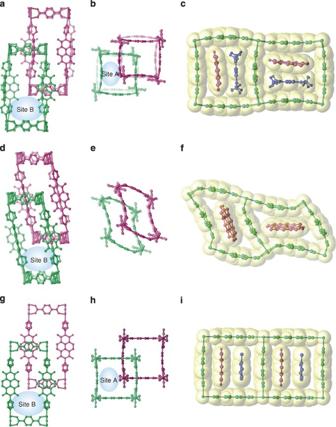Figure 3: Structural dynamics of1on the removal and incorporation of guest molecules. (a–c) The crystal structure of1a. The views along the main axes of bdc (a) and dpNDI (b) are shown. Site A is defined as the slit-type pore between dpNDI and bdc as shown in (b) and highlighted in (c). Site B illustrated in (a) presents the remaining pore. (d–f) The crystal structure of1b, determined after the removal of two DMF molecules from site A of1a. The grid composed of bdc and dpNDI is sheared while maintaining site B (d), and the shearing of the grid composed of two bdc units decreases the size of site A (e); this is also highlighted in (f). (g–i) The crystal structure of1c. The incorporation of toluene into1induces a structural transition to a non-distorted framework (g,h). Compared with1a(b), the displacement of one framework in the other, along the main axis of bdc, leads to an enlargement in the pore size of site A (h). The toluene molecule interacts with the NDI in site A in a face-to-face manner (i). One of the entangled frameworks is highlighted in green and the other in purple; the guest DMF and toluene molecules are shown in blue. The van der Waals surface is highlighted in yellow. Figure 3: Structural dynamics of 1 on the removal and incorporation of guest molecules. ( a – c ) The crystal structure of 1a . The views along the main axes of bdc ( a ) and dpNDI ( b ) are shown. Site A is defined as the slit-type pore between dpNDI and bdc as shown in ( b ) and highlighted in ( c ). Site B illustrated in ( a ) presents the remaining pore. ( d – f ) The crystal structure of 1b , determined after the removal of two DMF molecules from site A of 1a . The grid composed of bdc and dpNDI is sheared while maintaining site B ( d ), and the shearing of the grid composed of two bdc units decreases the size of site A ( e ); this is also highlighted in ( f ). ( g – i ) The crystal structure of 1c . The incorporation of toluene into 1 induces a structural transition to a non-distorted framework ( g , h ). Compared with 1a ( b ), the displacement of one framework in the other, along the main axis of bdc, leads to an enlargement in the pore size of site A ( h ). The toluene molecule interacts with the NDI in site A in a face-to-face manner ( i ). One of the entangled frameworks is highlighted in green and the other in purple; the guest DMF and toluene molecules are shown in blue. The van der Waals surface is highlighted in yellow. Full size image The novel entangled porous framework, [Zn 2 (bdc) 2 (dpNDI)] n ( 1 ) (bdc, 1,4-benzenedicarboxylate; dpNDI, N , N ′-di(4-pyridyl)-1,4,5,8-naphthalenediimide), was synthesized by mixing a solution of dpNDI and H 2 bdc with Zn(NO 3 ) 2 •6H 2 O in N , N -dimethylformamide (DMF) under solvothermal conditions. The crystals of 1 were obtained as 1 •4DMF ( 1a ), which incorporates four DMF molecules as guest molecules. As shown in Figure 3a–c , the single-crystal X-ray diffraction (SCXRD) measurements for 1a show that one of the frameworks of 1 was intergrown at the central position of the void that was created by the other framework. Notably, both dpNDI and bdc moieties are unusually bent to enhance the preferential π–π stacking interactions with an interframework distance of 3.35 Å along the two different directions of the Zn–bdc coordination modes. Therefore, two neighbouring dpNDI units exhibit almost perpendicular orientations ( Fig. 3c ). Here, the void spaces are classified as two different environments: the characteristic slit between dpNDI and bdc (site A, highlighted in Fig. 3c ) and the remaining void space (site B). Two DMF molecules occupy both sites A and B. Thermogravimetric (TG) analysis of 1a showed that DMF molecules were removed at 170 °C, and the resulting dried framework was stable up to 400 °C ( Supplementary Figs S1 and S2 ). The powder X-ray diffraction (PXRD) pattern changed markedly on the removal of DMF molecules and then returned to the original pattern of 1a after the sample was soaked in DMF ( Supplementary Fig. S3 ). The drying of a single 1a crystal in vacuum led to the formation of a single-crystal-to-single-crystal transition, generating 1 •DMF ( 1b ). The SCXRD analysis showed that the framework maintained its mutual position and interframework interaction; however, the framework had sheared itself to minimize the void spaces due to the removal of the DMF molecules at site A ( Fig. 3d–f ). One DMF molecule still occupied site B, in which the framework shearing did not significantly influence its size. Because the PXRD pattern of a fully dried sample of 1 corresponds to the simulation pattern of 1b , the distorted structure of 1b could be recognized as its dried structure ( Supplementary Fig. S4 ). The aromatic VOCs listed in Table 1 were successfully introduced into the entangled framework by immersion of a dry powder sample of 1 into the liquid of each aromatic VOC, which led the framework to accommodate each VOC ( 1 VOC ). Structural elucidation was successfully carried out with a guest-exchanged single crystal of 1 • 2.5toluene ( 1c ), which was prepared using the single-crystal-to-single-crystal transition of 1a to 1c in toluene. The SCXRD of 1c showed that a significant framework displacement on guest exchange had occurred; one framework slid along the main axis of one bdc molecule. Because the framework possessed two equivalent bdc molecules that were aligned in both the a - and b -axis directions (displacement can occur intrinsically along both directions, even in a single crystal), the crystallographic analysis was carried out on the basis of a pseudomerohedral twin crystal system. One of the twin structures is shown in Figure 3g–i . The characteristic bending of dpNDI and bdc in 1a was not observed in 1c ; all of the ligands changed to become planar. The framework displacement compensated for the bending of ligands to gain an interframework interaction between dpNDI and bdc (3.41 Å), with all of the dpNDI molecules aligned in one direction (along the a - or b -axis). Notably, one of the toluene molecules was strongly confined at site A ( Fig. 3i ), and this compound interacted with dpNDI in a face-to-face manner (3.6 Å). The PXRD patterns can be categorized into the following two main classes ( Supplementary Figs S5 and S6 ): those with XRD patterns identical to that of 1a for benzonitrile and anisole, and those with XRD patterns identical to that of 1c for the other methylated benzene compounds. This indicates that all methylated benzenes induced the same structural transformation as 1c and were trapped in the pores in a manner similar to that of toluene. Table 1 Properties of 1 VOCs. Full size table Molecular decoding by visualization of host–guest interactions The characteristic photophysical features of NDI allow for the implementation of a strategic decoding protocol. Because NDI interacts with aromatic VOCs and shows an exciplex emission that is modulated by a host–guest CT interaction, the emission wavelength, and therefore the emission colour, can be recognized as a readout that corresponds to the chemical substituent on the phenyl ring. Although several works have reported the synthesis and structure of PCPs with NDI derivatives, the photochemical properties of these compounds have not yet been described [37] , [38] , [39] , [40] , [41] , [42] . This can be attributed to the very weak fluorescent properties of NDI. The as-synthesized samples of 1a and the dried samples of 1 do indeed show a very weak fluorescence with a very low quantum yield ( Φ f <0.01) and a short average lifetime ( τ ∼ 150 ps). Therefore, we recognized this state as being a luminescence-off state. In contrast, because of the strong confinement at site A as a consequence of the framework displacement, a ground-state CT interaction between NDI and aromatic VOCs in all 1 VOC samples (except 1 benzonitirile , which has the lowest electron-donating ability in this series of VOCs) is observed as an additional broad absorption band at 420–500 nm ( Supplementary Fig. S7 ) and as the excitation spectra ( Supplementary Fig. S8 ). To date, this characteristic signature of the ground-state CT interaction has not been detected in solution studies [34] . The confinement effect enhances the CT characteristics. Therefore, all 1 VOC samples demonstrated fluorescence in the visible light region. 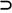Figure 4: Multicolour luminescence of1VOCs. (a) The resulting luminescence of crystal powders of1, suspended in each VOC liquid after excitation at 365 nm using a commercial ultraviolet lamp. (b) Height-normalized luminescent spectra of1VOCsafter excitation at 370 nm. (c) The relationship between the emission energy of1VOCsand the ionization potential of each VOC48. The linear correlation implies that the CT complexation dominates the fluorescence. Interestingly, the emission colour was dependent on the electronic structure of the VOCs used, as shown in Figure 4a . A new emission band after excitation at 370 nm for 1 toluene appeared at 476 nm with very high fluorescent intensity ( Φ f =0.22) and a long average lifetime ( τ ∼ 14.8 ns). Interestingly, the quantum yield reported here is ten times higher than that of a mixture of NDI derivatives and toluene in solution [34] . The emission wavelength, quantum yield ( Supplementary Fig. S9 ) and average lifetime ( Supplementary Fig. S10 and Supplementary Table S1 ) of the 1 VOCs , as well as the ionization potential of the VOCs, are summarized in Table 1 . The normalized emission spectra exhibited a gradual red shift as the electron-donating capability of VOCs increased after excitation of 1 VOCs at 370 nm ( Fig. 4b ). The following emissions were observed: 421 nm for 1 benzonitrile , 439 nm for 1 benzene , 476 nm for 1 toluene , 496 nm for 1 o -xylene , 503 nm for 1 m -xylene , 518 nm for 1 p -xylene and 592 nm for 1 anisole . This confirms that the CT complexation between NDI and VOCs contributed to the characteristic emission bands over the entire visible region (420–600 nm). The correlation of the fluorescence energy of 1 VOCs with the ionization potential of VOCs supports the significance of CT complexation ( Fig. 4c ). Figure 4: Multicolour luminescence of 1 VOCs . ( a ) The resulting luminescence of crystal powders of 1 , suspended in each VOC liquid after excitation at 365 nm using a commercial ultraviolet lamp. ( b ) Height-normalized luminescent spectra of 1 VOCs after excitation at 370 nm. ( c ) The relationship between the emission energy of 1 VOCs and the ionization potential of each VOC [48] . The linear correlation implies that the CT complexation dominates the fluorescence. Full size image Although the interframework interaction between NDI and bdc is significant in both 1a - and the 1c -type structures, it has no effect on the fluorescent properties. This is because of the low electron-donating ability of bdc, which is further reduced by coordination with zinc ions, producing very weak CT characteristics. Notably, the non-entangled analogue of 1 with 1,4-naphthalenedicarboxylate (ndc) as layer linkers, [Zn 2 (ndc) 2 (dpNDI)] n (ref. 43 ), demonstrates no fluorescence, even with the incorporation of toluene ( Supplementary Figs S11 and S12 ). This indicates that the framework entanglement is required to induce fluorescence based on CT complexation in this framework system. The framework incorporating methylated benzene with a 1c -type structure showed the highest fluorescent quantum yield ( Φ f =0.05–0.22). In addition, the 1a -type framework with either benzonitrile or anisole exhibited a significantly lower emission intensity ( Φ f ≤0.01) and a shorter average lifetime ( τ =0.3 or 5.6 ns, respectively), as summarized in Table 1 . This is most likely attributed to the framework structure and the electronic properties of the guest VOCs. The 1a -type structure cannot provide sufficient space at site A to exhibit efficient face-to-face interactions between NDI and VOCs, as shown in Figure 3c . In addition, the higher ionization potential of benzonitrile (IP=10.09 eV) does not provide sufficient electron-donating capabilities to permit CT complexation. In contrast, the strong donating property of anisole (IP=8.83 eV) may also quench the CT fluorescence by the contribution of the radical ion pair state, in which the total electron transfer from anisole to NDI deactivates the excited state by non-radiative decay. This radical ion pair state is most likely formed by introducing N , N -dimethylaniline, which demonstrates the strongest electron-donating properties (IP=7.12 eV). As soon as the dried sample of 1 was immersed into N , N -dimethylaniline ( Supplementary Fig. 13 ), the colour changed to purple. This occurred as a result of the broad absorption band observed at 500–600 nm ( Supplementary Fig. S14 ), followed by complete quenching of its fluorescence. This new absorption is ascribed to the radical form of NDI [44] , which was confirmed by well-defined electron paramagnetic resonance measurements ( Supplementary Fig. S15 ). Apart from the fluorescent decoding based on CT complexation described above, benzene substituted by a heavy atom (for example, iodine) led to a different type of emission mechanism. The 1 iodobenzene sample ( Supplementary Fig. S13 ) showed a characteristic red phosphorescence emission occurring at 640 nm ( Fig. 4a,b ) with a lifetime in the order of 100 μs ( τ =139 μs: Supplementary Fig. S16 and Supplementary Table S2 ), after excitation at 370 nm. It has been reported that, by mixing NDI and ethyl iodide in a glassy solvent at room temperature or under frozen conditions at 77 K, one can promote phosphorescence emission. This is thought to occur because the presence of a heavy atom that is situated very close to NDI favours the intersystem crossing from the excited π–π* singlet state to the close-lying n –π* triplet state [45] , [46] . Here, the effect of the strong confinement in the nanopores allows the heavy atom compound to lie in close proximity to NDI and enables a sufficient host–guest interaction to produce an effective population in the triplet state, even at room temperature. On the basis of a combination of these two mechanisms, exciplex emission with CT characteristics and phosphorescence, we succeeded in differentiating aromatic VOCs on the basis of their corresponding emission colour after simple excitation at 370 nm. Nonlinear response due to a cooperative structural transition As described above, the entangled framework shows a crystal-to-crystal structural transition from the dried phase of 1b to the guest accommodation phase of 1c , as well as the incorporation of an aromatic VOC molecule. In such a crystal-phase transition, the ordered framework structure in the mesoscopic crystal domain must be cooperatively transformed. In turn, a number of NDI-decoding units must be simultaneously accessible to the guest molecules (that is, the generation of site A in the 1c structure). Because the luminescent signal intensity is dependent on the number of CT interaction sites between NDI and VOC, the sensor response of 1 induced by a structural transition is expected to be nonlinear with respect to the concentration of the guest molecule. We carried out sensor response experiments by combining a vapour-control system with a fluorescent microscope equipped with a CCD camera ( Supplementary Fig. S17 ). A helium gas stream containing toluene vapour, the relative pressure of which was regulated using a mass-flow controller, was introduced into a quartz capillary containing crystals of the dried phase of 1 . 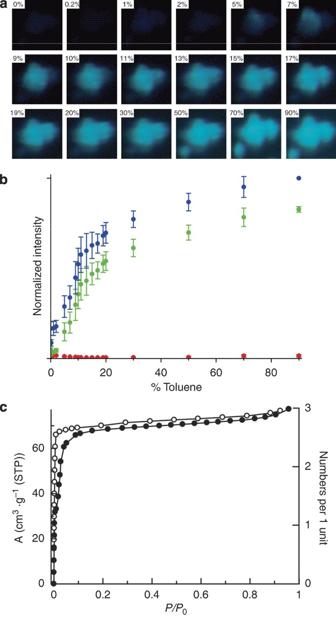Figure 5: Nonlinear fluorescent sensor response measurements of1at a controlled relative toluene vapour pressure. (a) A series of microscopic fluorescent images of1under the following relative toluene vapour pressures: 0, 0.2, 1, 2, 5, 7, 9, 10, 11, 13, 15, 17, 19, 20, 30, 50, 70 and 90%. (b) A plot of the RGB fluorescence intensity against the relative toluene vapour pressure in a helium gas stream showing the nonlinear sensor response of the blue and green signals. The data were obtained using the arithmetic mean of 14 samples. The error bars denote the standard deviation. (c) An adsorption isotherm of1for benzene with two adsorption steps with hysteresis clearly indicates the cooperative structural transformation in response to guest accommodation. The change in fluorescent intensity was imaged using the CCD camera under a microscope, as shown in Figure 5a . The dark state of 1 changed to the fluorescent 'turn-on' state of 1 toluene with increasing relative toluene vapour pressure. The emission colour of each fluorescent image was digitally converted into its RGB (red, green, blue) intensity. The RGB intensities obtained under the controlled relative toluene vapour pressure are plotted in Figure 5b . We carried out this experiment for 14 different powder crystals, and the average intensities and standard deviations are shown. The blue and green signals were detected as sensing outputs (cyan is the emission colour of 1 toluene ); however, the red signal was not detected. Interestingly, both blue and green signals showed nonlinear sensor responses. The sensing output increases markedly below a toluene dosage of 10%, after which the sensing output showed a gradual increase up to the saturation value at a relative toluene vapour pressure of 90%. It is worth noting that the intensity of the green signal was weak at very low relative pressures <2% and was almost identical to the dark background. This is most likely because of the toluene molecules that are initially accommodated at site B, in which the NDI moiety is not exposed. After the accumulation of a given number of guest molecules at site B, the framework changes its structure from 1b to 1c , leading to the accessibility of the NDI moiety for toluene and the emergence of emission based on the NDI–toluene interaction. Figure 5: Nonlinear fluorescent sensor response measurements of 1 at a controlled relative toluene vapour pressure. ( a ) A series of microscopic fluorescent images of 1 under the following relative toluene vapour pressures: 0, 0.2, 1, 2, 5, 7, 9, 10, 11, 13, 15, 17, 19, 20, 30, 50, 70 and 90%. ( b ) A plot of the RGB fluorescence intensity against the relative toluene vapour pressure in a helium gas stream showing the nonlinear sensor response of the blue and green signals. The data were obtained using the arithmetic mean of 14 samples. The error bars denote the standard deviation. ( c ) An adsorption isotherm of 1 for benzene with two adsorption steps with hysteresis clearly indicates the cooperative structural transformation in response to guest accommodation. Full size image The adsorption isotherm of the dried sample of 1 for benzene supports this phenomenon. We used benzene as a guest molecule, rather than toluene, because the higher boiling temperature of toluene restricts adsorption measurements at room temperature. As shown in Figure 5c , the two-step adsorption isotherm, with significant hysteresis at the low-vapour-pressure region, clearly indicates the cooperative structural transformation in response to benzene accommodation. Although the adsorption step was observed at lower vapour pressures, compared with the step in the luminescent sensor response measurement, this difference is most likely attributed to two significant differences in experimental conditions. Whereas benzene was used for the adsorption isotherm because of its low boiling point, toluene was chosen for the luminescent sensor response measurement because of its high quantum yield. Furthermore, the adsorption measurement was carried out by controlling the absolute vapour pressure of the analyte and by strictly estimating the equilibrium condition at each vapour pressure (hours for each point). In contrast, the sensor response measurement was taken with the analyte flow system in the carrier gas and by recoding 10 min intervals for each point. This molecular decoding strategy using luminescence is strongly correlated with the structural transformation dynamics in entangled frameworks. Regarding the electronic structure, size and shape of the guest molecules, the entangled framework [Zn 2 (bdc) 2 (dpNDI)] n demonstrates the displacement of two chemically non-interconnected frameworks, which provides space (site A) for trapping the guest molecule with an optimized host–guest interaction. Such a satisfactory confinement enhances the interaction of aromatic guest molecules with the NDI moiety embedded in the framework scaffolds. This leads to the formation of complexes with a CT nature, producing fluorescence from the exciplex, or the stabilization of the triplet state of NDI to generate phosphorescence. Because the luminescence from the optimized host–guest interaction is only dependent on the nature of the aromatic guest molecules (the ionization potential for the fluorescence and the heavy atom effect for the phosphorescence), the entangled framework system decodes the molecular information of the guest molecule by luminescence. In contrast, the dried structure of 1 was a significant structural phase when used as a sensor to trap the vapour of the guest molecule. In this dried structure, the framework sheared itself to minimize the void spaces that resulted in the elimination of site A. Because this structure is considered an initial state for the sensing experiment, it is expected that the structural transformation occurs in response to the guest molecule accommodation process. As the adsorption isotherm for benzene showed significant uptake in the very low pressure region ( P / P 0 <0.01), the dried framework accommodates benzene in site B ( Supplementary Fig. S18 ). Because site B is insignificant to exciplex formation, the green intensity arising from a characteristic cyan colour for the NDI-toluene exciplex fluorescence does not increase in the sensor response measurement. However, the step observed (near P / P 0 =0.02) in the adsorption isotherm implies that the cooperative structural transformation from the dried phase to the 1c -type structure allows guest molecules access to site A. Therefore, we observed a large increase in the green intensity in the sensor response measurement after the relative toluene pressure reached >2%, which resulted in a nonlinear sensor response. In this report, we have demonstrated a novel sensing method for distinguishing small structural differences in molecules using a sophisticated transduction protocol, molecular decoding. Information regarding different phenyl ring substituents of aromatic VOCs is decoded into a corresponding visible light emission and observed as a readout from the decoding matrix based on an NDI-embedded porous framework. Such a decoding protocol is observed by direct visualization of the host–guest interaction, either by exciplex emission based on the CT characteristics of the NDI and VOC or a phosphorescence-stabilized event based on a heavy atom that is attached to the aromatic guest. The aromatic guest molecules are strongly confined in the nanopores because of a dynamic structural transformation in the framework entanglement, and the resulting host–guest interaction produces an enhanced emission that is detectable by the naked eye. We have demonstrated that the cooperative structural transition induced by the adsorption of a guest molecule provides a nonlinear sensor response that can be used for the amplification of the signal intensity to achieve a high sensitivity. This simple yet sophisticated decoding method of combining a single excitation light wavelength and an RGB detector will enable new novel applications of crystalline porous materials as portable solid-state sensor devices. Materials All of the reagents used, except for dpNDI, were obtained from commercial suppliers and were used without further purification. The dpNDI was synthesized according to a previous report [47] . Preparation of {[Zn 2 (bdc) 2 (dpNDI)]·4(DMF)} n ( 1a ) A mixture containing Zn(NO 3 ) 2 •6H 2 O (149 mg, 0.50 mmol), H 2 bdc (83 mg, 0.50 mmol) and dpNDI (210 mg, 0.50 mmol) was suspended in DMF (50 ml) and heated to 95 °C for a period of 3 days. The slightly yellow crystals of 1a were then collected. Preparation of dried sample [Zn 2 (bdc) 2 (dpNDI)] n ( 1 ) The crystals of 1a were dried in a vacuum oven at 120 °C for 1 day, resulting in a dried framework, 1 . Elemental analysis of 1 calcd (%) for C 40 H 20 Zn 2 N 4 O 12 : C 54.63, H 2.29, N 6.37. Found: C 55.26, H 2.40, N 6.48. Preparation of 1 VOC Dried crystals of 1 were immersed in each VOC liquid for 1 week, resulting in the formation of 1 VOC . Measurements The TG analysis was carried out using a Rigaku Thermo plus TG 8120 apparatus (Rigaku) in the temperature range of 303–773 K under flowing N 2 gas at a heating rate of 10 K min −1 . Elemental analysis was carried out using a ThermoFinnigan EA 1112 apparatus. PXRD data were collected using a Rigaku RINT-2200 Right System (Ultima IV, Rigaku) diffractometer with CuKα radiation and at the BL13XU beamline (SPring-8) using a synchrotron X-ray source ( λ =1.55642 Å). The simulated patterns were obtained from single-crystal X-ray analysis. Ultraviolet–vis diffuse reflectance measurements were recorded using a JASCO V-670 spectrometer (JASCO) with an integration sphere attachment. The samples were dispersed in aluminium oxide (5 wt%). The excitation and fluorescence spectra were recorded using a suspension of the dispersed powder in the guest solvent, with a SPEX spectrofluorimeter equipped with a double monochromator in both the excitation and emission channels (HORIBA Fluorolog-3, HORIBA) and 1-cm quartz cuvettes. The emission and excitation spectra were recorded at 450 and 370 nm, respectively. The spectra were corrected for the monochromator wavelength dependence and photomultiplier response functions. Phosphorescence spectra were measured after excitation at 370 nm in a HORIBA Fluorolog-3 apparatus, using a flash lamp with a 50-μs delay after the flash and a gate time of 61 μs, accumulating 100 flash counts per point. The fluorescent and phosphorescent quantum yields were measured using an Absolute photoluminescence quantum yield measurement system (Hamamatsu, C9920-02). The radiative deactivation curves for the fluorescence were recorded using a Time-correlated single-photon counting technique (Edinburgh Instruments, model FL 920) with a time resolution of 30 ps after deconvolution of the excitation pulse. Excitation was performed using Diode lasers (PicoQuant, model LDH 370), using a pulse with a full-width at half-maximum of 150 ps and a repetition rate of 2,500 kHz. The data were recorded at the emission maximum of each sample. The samples were measured in a suspension of dispersed powder in the guest solvent. The radiative deactivation curve of the phosphorescence was recorded using a HORIBA FluoroCube (HORIBA). Excitation was carried out using a SpectraLED-370. Data were recorded at the emission maximum of 635 nm. Electron spin resonance spectra were recorded at 77 K using a JEOL JES-RE2X spectrometer (JEOL) operating in the X-band. Resonance frequency was measured using an ADVANTEST R5372 microwave frequency counter (ADVANTEST). Sorption isotherm measurements were recorded using an automatic volumetric adsorption apparatus (BELSORP-max; BEL Japan). The as-synthesized samples were evacuated under high vacuum (<10 −2 Pa) at 393 K overnight to remove guest molecules. The adsorbate was placed into the sample tube and, before measurement, evacuated again using the degas function of the analyser for 2 h at 393 K. The change in pressure was monitored, and the degree of adsorption was determined by the decrease in pressure at the equilibrium state. SCXRD measurements of 1a –– 1c Single crystals of 1a – 1c were mounted in a loop. Measurements were taken using a Rigaku AFC10 diffractometer using a Rigaku Saturn CCD system (Rigaku) equipped with a rotating anode X-ray generator that produced multilayer mirror monochromated MoKα radiation. In all cases, the structure was elucidated using direct methods and refined using full-matrix least-squares techniques on F 2 (SHELXL-97). All of the non-hydrogen atoms were anisotropically refined, whereas all hydrogen atoms were placed geometrically and refined using a riding model with U iso constrained to be 1.2 times U eq of the carrier atom. The crystal of 1c was a pseudomerohedral twin, and the refinement against the intensities was carried out using the SHELXL-97 software package, including the twinning operator ( k , h , l ) (TWIN) as the twin fraction (batch scale factor, initially set to 0.5). The twin component of the final material comprised 66.18% of the crystal. The number of toluene molecules was determined by thermogravimetric measurements: 2.5 toluene molecules per two Zn atoms. The two guest toluene molecules were initially generated by fixing the bond length to 1.35 Å, the bond angle to 120° and the torsion angle to 0°. The remaining 0.5 toluene molecule was highly disordered; further refinement was unsuccessful. All parameters were refined by restraining these values and the thermal factors. Crystallographic data for 1a , 1b and 1c ( Supplementary Data S1 , 2 , 3 ) have been deposited in the Cambridge Crystallographic Data Center under deposition numbers CCDC 743922, 773586 and 743923, respectively. Sensor response as a function of toluene vapour pressure Sensor response measurements were taken using a Fluorescent microscope (BX 51, Olympus) with a 100-W mercury lamp (USH-1030L, Olympus) connected to a BEL-Flow vapour control system (BEL Japan). A schematic illustration of this system is shown in Supplementary Fig. S17 . The light source was filtered using an excitation filter that had a light transmission bandwidth between 330 and 385 nm (U-MWU2, Olympus), as well as neutral density filters (U-25ND25 and U-25ND6, Olympus). The fluorescence above 400 nm was detected using a CCD camera (DP72, Olympus) with a 30 ms exposure time. The relative toluene vapour pressure in a helium gas stream was controlled using three independent mass flow controllers in the range of 0.0–90.0%. The toluene vapour saturated carrier gas was generated by passing it through toluene (28 °C) and cooling it to 25 °C using a condenser. The toluene-saturated gas was then mixed with dry helium gas to obtain the desired relative pressure. The vapour gas flowed into a quartz capillary that contained the sample for a period of 10 min at a flow rate of 100 cm 3 min −1 . How to cite this article: Takashima, Y. et al . Molecular decoding using luminescence from an entangled porous framework. Nat. Commun. 2:168 doi: 10.1038/ncomms1170 (2011).